Evidence for massive bulk Dirac fermions in Pb1−xSnxSe from Nernst and thermopower experiments Topological surface states protected by mirror symmetry are of interest for spintronic applications. Such states were predicted to exist in the rocksalt IV–VI semiconductors, and several groups have observed the surface states in (Pb,Sn)Te, (Pb,Sn)Se and SnTe using photoemission. An underlying assumption in the theory is that the surface states arise from bulk states describable as massive Dirac states, but this assumption is untested. Here we show that the thermoelectric response of the bulk states displays features specific to the Dirac spectrum. By relating the carrier density to the peaks in the quantum oscillations, we show that the first ( N =0) Landau level is non-degenerate. This finding provides robust evidence that the bulk states are indeed massive Dirac states. In the lowest Landau level, S xx displays a striking linear increase versus magnetic field characteristic of massive Dirac fermions. In addition, the Nernst signal displays a sign anomaly in the gap-inverted phase at low temperatures. The rocksalt IV–VI semiconductors have been identified by Fu et al. [1] , [2] as a novel class of insulators—the topological crystalline insulators—which display surface states that are protected by crystalline symmetry. The topological surface states in topological crystalline insulators are to be contrasted with those in the widely investigated Z2 invariant topological insulators, which are protected by time-reversal invariance [3] , [4] . Angle-resolved photoemission spectroscopy (ARPES) experiments have obtained evidence for the surface states in Pb 1− x Sn x Se (ref. 5 ), SnTe (ref. 6 ) and Pb 1− x Sn x Te (ref. 7 ). In the alloys Pb 1− x Sn x Te and Pb 1− x Sn x Se, the bulk electrons occupy four small Fermi surface (FS) pockets located at the L points in k space (inset, Fig. 1 ). The conduction band is predominantly derived from the cation Pb 6 p orbitals, whereas the uppermost valence band is predominantly anion 4 p (or 5 p ) orbitals (ordering similar to the atomic limit) [8] . As the Sn content x increases, the system undergoes gap inversion when x exceeds a critical value x c (refs 9 , 10 , 11 , 12 ). In samples with x ≥ x c , gap inversion occurs when the temperature T is lowered below the gap-inversion temperature T inv . The ARPES experiments [5] , [6] , [7] confirm that the predicted topological surface states appear in the gap-inverted phase. 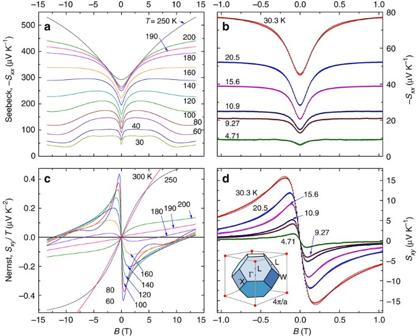Figure 1: Thermopower and Nernst effect in a topological crystalline insulator. The panels provide an overview of how the thermopowerSxxand Nernst signalSxyvary with fieldBin a high-mobility crystal (sample 1) of Pb1−xSnxSe withx=0.23. (a,b) Curves ofSxxversusBat selectedT(sample 1). At eachT, theV-profile bracketingB=0 reflects the rapid crossover from smallμBto largeμBregime. (c) The Nernst signalSxy/Tfrom 60 to 300 K. The sharp peaks reflect the semiclassical response. An anomalous sign change occurs atTinv=180 K. (b,d) Fits equations 1 and 2 (thin curves) toSxxandSxyat lowB. ForSxy(d), we have had to invert the sign. At 30.3 K, the best-fit values ofμ, andHare 51,404 cm2V−1s−1, 61.5 eV−1and 104.6 eV−1, respectively. At 4.71 K, the corresponding values are 113,250cm2V−1s−1, 52.3 eV−1and 81.3 eV−1. The inset shows theL(111) points on the hexagonal faces of the Brillouin Zone. Figure 1: Thermopower and Nernst effect in a topological crystalline insulator. The panels provide an overview of how the thermopower S xx and Nernst signal S xy vary with field B in a high-mobility crystal (sample 1) of Pb 1− x Sn x Se with x =0.23. ( a , b ) Curves of S xx versus B at selected T (sample 1). At each T , the V -profile bracketing B =0 reflects the rapid crossover from small μB to large μB regime. ( c ) The Nernst signal S xy / T from 60 to 300 K. The sharp peaks reflect the semiclassical response. An anomalous sign change occurs at T inv =180 K. ( b , d ) Fits equations 1 and 2 (thin curves) to S xx and S xy at low B . For S xy ( d ), we have had to invert the sign. At 30.3 K, the best-fit values of μ , and H are 51,404 cm 2 V −1 s −1 , 61.5 eV −1 and 104.6 eV −1 , respectively. At 4.71 K, the corresponding values are 113,250cm 2 V −1 s −1 , 52.3 eV −1 and 81.3 eV −1 . The inset shows the L (111) points on the hexagonal faces of the Brillouin Zone. Full size image The new topological ideas invite a fresh look at the bulk states of the IV–VI semiconductors. To date, the gap inversion appears to have no discernible effect on transport properties (the resistivity, Hall coefficient and thermopower vary smoothly through T inv ). This is surprising given that transport probes the states at the Fermi level. Moreover, a long-standing prediction [8] , [13] is that the bulk electrons occupy states described by the massive Dirac Hamiltonian. This assumption underlies the starting Hamiltonian of Hsieh et al. [2] However, no experimental test distinguishing the massive Dirac from the Schrödinger Hamiltonian has appeared to our knowledge. We have grown crystals of Pb 1 − x Sn x Se ( x =0.23) in which the n -type carriers have high mobilities ( μ =114,000 cm 2 V −1 s −1 at 4 K). The low electron density (3.46 × 10 17 cm −3 ) enables the quantum limit to be reached at 7.7 T (measurements reveal that holes are absent). In addition to resistivity, we have used both thermopower and the Nernst effect to probe the states in fields up to 34 T. Surprisingly, the Nernst signal is observed to change its sign at T inv . To date, this appears to be the only transport or thermodynamic quantity that is strongly affected by gap inversion. In a thermal gradient and an applied magnetic field , the diffusion of carriers produces an electric field E , which is expressed as the thermopower signal S xx =− E x /| ∇ T | and the Nernst signal S xy = E y /| ∇ T |. In the semiclassical regime, the Mott relation [14] simplifies S xx and S xy to the form (see Methods section) where . The dependence on B appears only in the conductivity matrix elements σ ij ( B ) (for brevity, we write σ ≡ σ xx ). The parameters =∂ln σ /∂ζ and H =∂lnσ xy /∂ζ are independent of the mobility μ ( ζ is the chemical potential). Equation 1 describes the crossover in S xx from (at B =0) to H when μB >>1. Correspondingly, S xy increases linearly from 0 to peak at the value 1/2( H −) at B =1/ μ before falling as 1/ B when μB >>1. For n -type carriers, both and σ xy are negative, and S xx <0. From equation 2, the Nernst signal S xy is positive if H > (we discuss the sign convention in the Methods section). In terms of the exponents β and β H defined by σ ( E )~ E β and σ xy ~ E β H , we have = β / E F and H = β H / E F . Even for one-band systems, equations 1 and 2 have not received much experimental attention, possibly because real materials having only a single band of carriers with a low density (and high mobility) are rare. The analysis of S ij is complicated by the extreme anisotropy of the FS pockets in many semi-metals. For recent Nernst measurements on Bi and Bi 2 Se 3 , see refs 15 , 16 . For results on S ij in graphene, see refs 17 , 18 , 19 . The angular variation of the SdH period in Bi is investigated in refs 20 , 21 . In the annealed crystals of Pb 1− x Sn x Se (with x ~ x c ) investigated here, our measurements reveal only n -type carriers (holes are absent). The FS pockets are very small (the quantum limit is reached at 7.7 T) and nearly isotropic (as shown by field-tilt measurements). We find that equations 1 and 2 provide a very good fit to S xx and S xy in the semiclassical regime. Here we provide evidence that the bulk electronic states at the L points are in fact massive Dirac states. A characteristic feature of the massive Dirac spectrum is that in a magnetic field, the lowest Landau level (LL) is non-degenerate with respect to the spin degrees, whereas all higher LLs are doubly degenerate. Knowing the carrier density, we show that the field at which the chemical potential jumps to the lowest LL accurately determines its spin degeneracy to be 1. This confirms the starting assumption of ref. 2 . The unusual thermoelectric response is also investigated deep in the quantum limit. In addition, we show that the sign of the Nernst signal is anomalous (relative to standard Boltzmann theory) within the gap-inverted phase. Semiclassical regime Figure 1a-1b plots curves of the thermopower S xx versus B for selected T . From 250 to 160 K, the dominant feature is the rapid increase in weak B followed by saturation to a B -independent plateau at large B . As noted, the Nernst signal (shown as S xy / T in Fig. 1c ) changes from positive to negative as T is decreased below 180 K (identified with T inv ). As shown in Fig. 1b , the curves of S xx versus B fit very well to equation 1 in the semiclassical regime (| B |<1T). Likewise, below 100 K the curves of S xy also fit well to equation 2 up to an overall sign ( Fig. 1d ). Although the fit parameters ( μ , , H ) for S xx are independent of those for S xy , we find that they agree with each other (at the level of ±2%) below 60 K (see Methods section). At each T , the two curves, S xx ( B ) and S xy ( B ), are described by just three parameters. This provides a potent self-consistency check of equations 1 and 2. As a further test, we have also fitted the measured conductivity tensor σ ij ( B ) and obtained similar values for μ below 100 K (Methods). By and large, the close fits to both tensors S ij and σ ij demonstrate that we have one band of carriers below 100 K. The semiclassical expressions are no longer valid when quantum oscillations appear at higher B . In particular, the giant step at 7.7 T in the curves at 30 and 40 K ( Fig. 1a ) is a relic of the quantum regime that remains resolvable up to 100 K. The step has a key role in the discussion later. In the opposite extreme above 100 K, the two sets of fit parameters begin to deviate. The disagreement is especially acute near 180 K, where S xy changes sign. We reason that the one-band assumption breaks down because of strong thermal activation of holes as the gap closes and re-opens across T inv . The evidence comes from the T dependence of the Hall density n H = B / eρ yx (solid circles in Fig. 2a ). Whereas n H is nearly T -independent below 80 K, in agreement with the one-band model, it deviates upwards above 180 K. Thermal activation of a large population of holes leads to partial cancellation of the Hall E -field and a reduction in | ρ yx |. 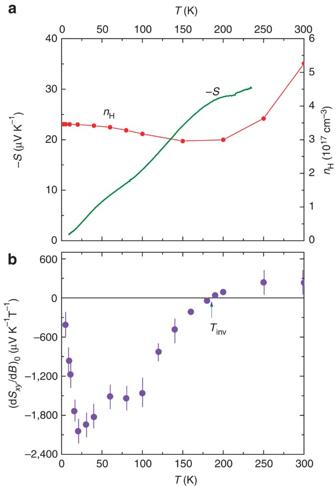Figure 2: Temperature dependence of Hall density, thermopower and Nernst slope. (a) TheTdependence of the Hall densitynH=B/ρyxeinferred from the Hall resistivityρyxand the zero-BthermopowerS(T)≡Sxx(T,B=0) in Pb1−xSnxSe (x=0.23). The Hall signal isn-type at allT. Below 20 K,nHequals 3.46 × 1017cm−3(sample 1).nHincreases significantly above 200 K signalling thermal activation of holes across the band gap. (b) TheTdependence of the initial slope of the Nernst signaldSxy/dB(B→0) to show the sign change atTinv. The error bars correspond to 1 s.d. in determiningdSxy/dBin the limitB→0. Figure 2: Temperature dependence of Hall density, thermopower and Nernst slope. ( a ) The T dependence of the Hall density n H = B / ρ yx e inferred from the Hall resistivity ρ yx and the zero- B thermopower S ( T )≡ S xx ( T , B =0) in Pb 1− x Sn x Se ( x =0.23). The Hall signal is n -type at all T . Below 20 K, n H equals 3.46 × 10 17 cm −3 (sample 1). n H increases significantly above 200 K signalling thermal activation of holes across the band gap. ( b ) The T dependence of the initial slope of the Nernst signal dS xy / dB ( B →0) to show the sign change at T inv . The error bars correspond to 1 s.d. in determining dS xy / dB in the limit B →0. Full size image In Fig. 2a , we have also plotted the zero- H thermopower S≡S xx (0) to bring out its nominally T -linear variation below 100 K (bold curve). The large value of the slope S(T)/T =1.41 μV K −2 implies an unusually small E F . As discussed, the Nernst signal changes sign at T inv =180 K. The T dependence of its initial slope dS xy /dB ( B →0) is displayed in Fig. 2b . From the fits to equations 1 and 2, we may address the interesting question whether the sign anomaly occurs in the gap-inverted phase ( T<T inv ) or in the uninverted phase. On both sides of T inv , the fits of S xx imply H > (that is, | S xx | always increases as μB goes from 0 to values >>1). As S xy ~( H −), we should observe a positive S xy . Hence, the sign anomaly occurs in the gap-inverted phase (in Fig. 1d , we multiplied the curves by an overall minus sign). The sign of the Nernst signal below T inv disagrees with that inferred from equations 1 and 2, despite the close fit. Further discussion of the sign anomaly is given below (see Discussion section). However, we note that the sign of S xy is independent of the carrier sign. As seen in Fig. 2a , both S and n H vary smoothly through T inv without a sign change. Quantum oscillations As shown in Fig. 3 , oscillations in S xx and S xy grow rapidly below 60 K to dominate the weak- B semiclassical profile. The most prominent feature in S xx is the large step decrease at the field B 1 =7.7 T (at which the chemical potential ζ jumps from the N =1 LL to the N =0 LL). In the Nernst curves, plotted as S xy / T in Fig. 3b , the quantum oscillations are more sharply resolved. As S xy is the off-diagonal term of the tensor S ij , its maxima (or minima) are shifted by 1/4 period relative to the extrema of the diagonal S xx (analogous to the shift of σ xy relative to σ ). This shift is confirmed in Fig. 4a , which plots the traces of S xx and S xy versus 1/ B . For the analysis below, we ignore the weak spin splitting, which is resolved in the N =1 LL (and barely in N= 2). 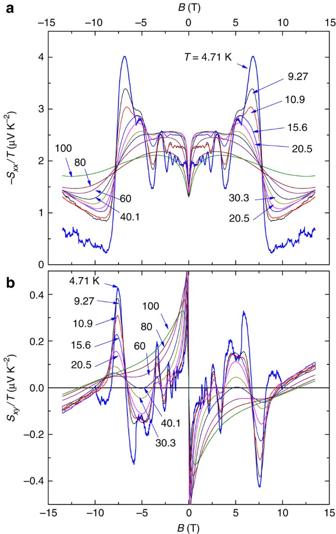Figure 3: Quantum oscillations in the thermopower and Nernst signal of PbSnSe. (a) Curves ofSxx/TversusBatT=4.71 to 100 K of Pb1−xSnxSe (x=0.23, sample 1). |Sxx/T| displays a maximum whenζis at the DOS maximum in each LL. At 4.71 K, theN=1 LL (5–7 T) displays a weak spin splitting. The giant step at 7.7 T occurs whenζenters theN=0 LL. (b) Curves ofSxy/Tfor the sameT. The sharp resonance-like peaks at low fields are the semiclassical response of largeμelectrons. Below 30 K, they are eclipsed by strong quantum oscillations. Figure 3: Quantum oscillations in the thermopower and Nernst signal of PbSnSe. ( a ) Curves of S xx / T versus B at T =4.71 to 100 K of Pb 1− x Sn x Se ( x =0.23, sample 1). | S xx / T | displays a maximum when ζ is at the DOS maximum in each LL. At 4.71 K, the N =1 LL (5–7 T) displays a weak spin splitting. The giant step at 7.7 T occurs when ζ enters the N =0 LL. ( b ) Curves of S xy / T for the same T . The sharp resonance-like peaks at low fields are the semiclassical response of large μ electrons. Below 30 K, they are eclipsed by strong quantum oscillations. 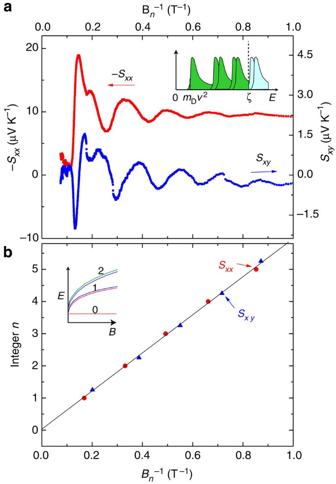Figure 4: Analysis of the quantum oscillations. (a) Comparison of curves ofSxxandSxyversus 1/Bat 4.71 K in Pb1−xSnxSe (x=0.23). The maxima inSxyare shifted by aperiod relative to the maxima inSxx. TheN=1 LL shows a weak spin splitting. The sketch (inset) shows the peaks in the DOS of each LL for 3D massive Dirac fermions. (b) Index plot ofBncorresponding to the maxima in |Sxx| (solid circles) andSxy(triangles) versus the integersn. The straight line is the relationF=2π(n+γ)/whereFis the FS section andγthe Onsager phase. The maxima inSxyare shifted byinn. From the slope, we infer the Fermi wavevectorkF=0.0134 Å−1andne=8.20 × 1016cm−3(per valley). The inset shows the LL energyEversusBin the massive Dirac spectrum forkz=0 (ref.22). Full size image Figure 4: Analysis of the quantum oscillations. ( a ) Comparison of curves of S xx and S xy versus 1/ B at 4.71 K in Pb 1− x Sn x Se ( x =0.23). The maxima in S xy are shifted by a period relative to the maxima in S xx . The N =1 LL shows a weak spin splitting. The sketch (inset) shows the peaks in the DOS of each LL for 3D massive Dirac fermions. ( b ) Index plot of B n corresponding to the maxima in | S xx | (solid circles) and S xy (triangles) versus the integers n . The straight line is the relation F =2 π ( n + γ )/ where F is the FS section and γ the Onsager phase. The maxima in S xy are shifted by in n . From the slope, we infer the Fermi wavevector k F =0.0134 Å −1 and n e =8.20 × 10 16 cm −3 (per valley). The inset shows the LL energy E versus B in the massive Dirac spectrum for k z =0 (ref. 22 ). Full size image Figure 4b shows the index plot of 1/ B n (inferred from the maxima in | S xx | and S xy ) plotted versus the integers n . From the slope of the line, we derive the FS section S F =5.95 T=5.67 × 10 16 m −2 . Assuming a circular cross-section, we have k F =0.0134 Å −1 . The electron concentration per FS pocket is then =8.2 × 10 16 cm −3 . As there are four pockets, the total carrier density is 4 n e =3.28 × 10 17 cm −3 , in good agreement with the Hall density n H at 4 K (3.46 × 10 17 cm −3 ). Using sample 2, we have tracked the variation of the SdH period versus the tilt angle θ of B . 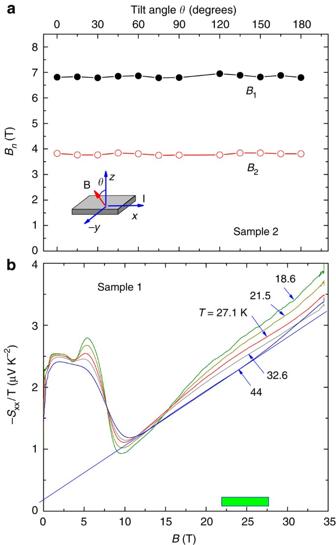Figure 5: Dependence of SdH period on field-tilt angle and high-field thermopower. (a) The dependence of the transition fieldsB1andB2versus tilt angleθofBin sample 2 (x=0.23) inferred from magnetoresistance (B1andB2are the fields at whichζjumps from LL withN=1→0 andN=2→1, respectively). Within our resolution, no angular dependence ofB1andB2is observed.Bis rotated in they–zplane (sketch in inset). (b) High-field measurements ofSxx/Tto 34 T at severalTin sample 1. TheB-linear dependence smoothly extends through the region 22–28 T where the transition (0, −)→(0, +) should have appeared. The interval 22–28 T is indicated by the horizontal green bar. Figure 5a plots the fields B 1 and B 2 versus θ ( B is rotated in the y – z plane). Here, B 1 and B 2 are the fields at which ζ jumps from N =1→0 and from N =2→1, respectively. To our resolution, the SdH period is nearly isotropic. The fields B 1 and B 2 are also independent of tilt angle when B is rotated in the x – y plane. This justifies treating the FS pockets as nominally spherical. Figure 5: Dependence of SdH period on field-tilt angle and high-field thermopower. ( a ) The dependence of the transition fields B 1 and B 2 versus tilt angle θ of B in sample 2 ( x =0.23) inferred from magnetoresistance ( B 1 and B 2 are the fields at which ζ jumps from LL with N =1→0 and N =2→1, respectively). Within our resolution, no angular dependence of B 1 and B 2 is observed. B is rotated in the y – z plane (sketch in inset). ( b ) High-field measurements of S xx / T to 34 T at several T in sample 1. The B -linear dependence smoothly extends through the region 22–28 T where the transition (0, −)→(0, +) should have appeared. The interval 22–28 T is indicated by the horizontal green bar. Full size image The N =0 Landau level We next address the question whether the bulk states in the inverted phase are Dirac fermions or Schrödinger electrons. The two cases differ by a distinctive feature in their LL spectrum that is robust against small perturbations. In the quantum limit, the massive Dirac Hamiltonian exhibits an interesting twofold difference in degeneracy between the N =0 and N =1 levels. Wolff [22] considered a three-dimensional (3D) massive Dirac Hamiltonian with spin–orbit interaction but no Zeeman energy term. More recently, Serajedh et al. [23] included the Zeeman energy term as well as a Rashba term in the massive two-dimensional (2D) Dirac Hamiltonian. Other 3D massive Dirac cases are discussed by Bernevig and Hughes [24] . All these authors find that N =0 LL is non-degenerate with respect to spin degrees, whereas the LLs with N ≠0 are doubly spin degenerate (we discuss in Methods section a pedagogical example, which shows that this anomaly is related to the conservation of states). By contrast, for the Schrödinger case, all LLs are doubly degenerate. In Pb 1− x Sn x Se, the ability to measure accurately both n e and the ‘jump’ field B 1 provides a crisp confirmation of this prediction. The energy of the N th LL is , where m D is the Dirac mass and the magnetic length [24] . At B 1 , E F lies just below the bottom of the N =1 LL so that all the electrons are accomodated in the N =0 LL. Integrating the density of states (DOS) for one spin polarization in the N =0 LL from m D v 2 to E F , we find (see Methods section) Ignoring the small spin splitting, we equate B 1 with 7.7 T. Equation 3 then gives n e↑ =9.0 × 10 16 cm −3 , which agrees within 10% with the measured n e (the agreement is improved if we correct for spin splitting). All the electrons are accomodated by an N =0 LL that is non-degenerate, in agreement with the prediction for massive Dirac states [22] , [23] , [24] , but disagreeing with the Schrödinger case by a factor of 2. As the singular spin degeneracy of the N =0 LL cannot be converted to a double degeneracy, the experiment uncovers a topological feature of the bulk states that is robust. As predicted in refs 22 , 23 , 24 , the N =0 LL has only one spin state (0,+); the spin-down partner (0,−) is absent. To check this further, we extended measurements of S xx to 34 T to search for the transition from the sublevel (0,−) to (0,+) (which should occur if N =0 LL were doubly degenerate). From extrapolation of the spin split N =1 and N =2 LLs, we estimate that the transition (0,−)→(0,+) should appear in the interval 22–28 T. As shown in Fig. 5b , the measured curves show no evidence for this transition to fields up to 34 T. Finally, we note an interesting thermopower feature in the quantum limit. At fields above B 1 , S xx displays a B -linear profile that extends to 34 T ( Fig. 5 ). The B -linear behaviour is most evident in the curve at 44 K. As T is decreased to 18.6 K, we resolve a slight downwards deviation from the linear profile in the field interval 10–20 T. The B -linear profile appears to be a characteristic property of massive Dirac fermions in the quantum limit. We discuss below a heuristic, semiclassical approach that reproduces the observed profile. We summarize the electronic parameters inferred from our experiment and relate them to ARPES measurements. As noted, the FS section derived from the index plot ( Fig. 4b ) corresponds to a total electron density 4 n e =3.28 × 10 17 cm −3 , in good agreement with the Hall density n H at 4 K (3.46 × 10 17 cm −3 ). We may estimate E F from the slope of the thermopower S(T)/T =1.41 μV K −2 . Using the Mott expression S(T) =( π 2 /3)( k B / e )( k B T / E F ) β , we find for the Fermi energy E F =17.0 β meV. For the massive Dirac dispersion, we have , which implies that β has the minimum value 3 (if the mobility increases with E , β is larger). Using the lower bound, β =3, S/T gives E F =51 meV. These numbers may be compared with ARPES measurements. We estimate the Fermi velocity from the expression v ~ E F / ħk F (valid when E F ≫ m D v 2 with m D the Dirac mass). Using our values of E F and k F , we find v =5.74 × 10 5 m s −1 as the lower bound. Although ARPES experiment cannot resolve v in the conduction band, the ARPES estimate [5] for the hole band velocity is 5.6 × 10 5 m s −1 , in good agreement with our lower bound. It is likely to be that the conduction band has a higher velocity (which would then require β >3). One of our findings is that gap inversion changes the sign of the Nernst signal. As the energies of states involved in gap inversion are very small, the resulting dispersion can be hard to resolve by ARPES measurement. Transport quantities would appear to be more sensitive to these changes. As noted, however, most transport quantities are either unaffected or only mildly perturbed. The Hall effect and thermopower are unchanged in sign across T inv ( Fig. 2a ). Although n H shows a gradual increase, this is largely attributed to thermal activation of holes across a reduced gap for T > T inv . Hence, the dramatic sign change observed in S xy stands out prominently; its qualitative nature may provide a vital clue. It has long been known [10] that in the lead rocksalt IV–VI semiconductors, the energy gap E g undergoes inversion as the Sn content x increases from 0. Moreover, within a narrow range of x , gap inversion is also driven by cooling a sample (the critical temperature is x dependent within this interval). Strauss [10] performed early optical transmission measurements of E g in a series of single-crystal films of Pb 1− x Sn x Se, with x ranging from 0 to 0.35. For x= 0.25, he reported that E g closes at 195 K. A slight interpolation of his data shows that at our doping x= 0.23, E g should vanish at 179 K, remarkably close to our T inv =180 K. The recent ARPES measurements of Dziawa et al. [5] is consistent with E g closing between 100 and 200 K. Given the ARPES resolution, these results are all consistent with our inference that our T inv corresponds to the gap inversion temperature. Hence, we reason that the Nernst signal changes sign either at, or very close to, the gap inversion temperature. The inverted sign of S xy below 180 K in Fig. 1c,d occurs in the gap-inverted phase. We refrain from making the larger claim that this is also the topological transition because we are unable to resolve the surface states in our experiments. The fits of S xy to equation 2 ( Fig. 1d ) shows that the curves below 100 K are well described by the Boltzmann–Mott expression assuming a single band of carriers, but there is an overall sign disagreement. Despite the sign problem, the analysis singles out the physical factors that fix the sign and delineates the scope of the problem. For example, reversing the sign of both β and β H inverts the sign of S xy , but also that of S xx . Alternately, one might try reversing the signs of β and β H , and e simultaneously. This will invert the sign of S xy but leave S xx unchanged. However, ρ yx is forced to change sign. The analysis assumes that in the gap-inverted phase, the FS is simply connected. This may not be valid. Gap inverion may lead to the existence of a small pocket surrounded by a larger FS sheet (topologically similar to the FS of the ‘giant Rashba’ material BiTeI [25] ). As the small pocket dominates the thermoelectric response, the Nernst effect may be detecting this novel situation. These issues will be left for future experiments. We may attempt to understand the striking B -linear profile of S xx / T in Fig. 5 using a semiclassical approach. In N =0 LL, the long-lived quasiparticles complete a large number of cyclotron orbits between scattering events (for example, from μB ~220, we estimate this number is ~35 at 20 T). The scattering results in the drift of the orbit centres X in a direction transverse to the applied − ▿ T . Ignoring the fast cyclotron motion, we may apply the Boltzmann equation to X . The thermopower is then given by the high- B limit of equation 1, S xx ( T , H )→ β H ′/ E F , where E F is now measured from the bottom of N =0 LL and β H ′ differs from the weak-field β H . In this picture, the B dependence of S xx arises solely from how E F changes with B . For B > B 1 , only N =0 LL is occupied. From equation 14 (Methods), we have the relation between E F , n e and B , viz. In the limit E F ≫ m D v 2 , we obtain the relation E F ~1/ B . This immediately implies that S xx / T increases linearly with B as observed. Setting g s =1, we derive from equation 4 the rate of increase Repeating this calculation for the Schrödinger case, we get instead S xx / T~B 2 . From Fig. 5 , the thermopower slope ∂( S xx / T )/∂( B )=8.71 × 10 −8 V K −2 T −1 . Using the above values of v and n e in equation 5, we find (∂ S xx / T )/∂( B )=6.1 β ′ H × 10 −8 V K −2 T −1 . The value of β ′ H is not known. Comparison of the calculated slope with experiment suggests β ′ H ~1.5. Hence, this back-of-the-envelop estimate can account for the rate at which S xx / T increases with B . Semiclassical fits to S xx and S xy In the presence of a magnetic field B , an electric field E and a temperature gradient − ∇ T (in an infinite medium), the total current density is given by [14] J = σ · E + α ·(− ∇ T ). Here, σ ij is the conductivity tensor and α ij is the thermoelectric tensor. Setting J =0 (for a finite sample) and solving for E , we have E =− ρ · α ·(− ∇ T ), with ρ = σ −1 the resistivity tensor. In the geometry with and , the components of the E -field (for an isotropic system) are The thermoelectric tensor S ij is given by E i = S ij ∂ j T ( S xx >0 for hole carriers and S xy >0 if E y >0 when H z >0). The Mott relation [14] , where k B is Boltzmann’s constant, e is the elemental charge and ζ the chemical potential, has been shown to hold under general conditions, for example, in the quantum Hall Effect (QHE) [26] , [27] . Using equation 8, equations 6 and 7 reduce to equations 1 and 2, respectively. The fits of S ij to these equations displayed in Fig. 1d were carried out using the one-band, Boltzmann–Drude expressions for the conductivity tensor, viz. where the total carrier density N e is 4 n e ( n e is the density in each of the FS pocket at the L points). In the geometry with and , we define the sign of the Nernst signal to be that of the y component of the E -field E y . More generally, if E N is the E -field produced by the Nernst effect, the sign of the Nersnt signal is that of the triple product E N · B × (− ∇ T ). This agrees with the old convention based on ‘Amperean current’ [28] and with the one adopted for vortex flow in superconductors [29] . At each T , we have fitted the measured curves of S xx and S xy versus B to equations 1 and 2 using equations 9 and 10 for the conductivity tensor. The separate fits of S xx and S xy yield two sets of the parameters μ , and H , which are displayed in Fig. 6 (solid triangles and open circles, respectively). The three-parameter fit places strong constraints on the curves of S xx and S xy . Disagreement between the two sets signals that the one-band model is inadequate. 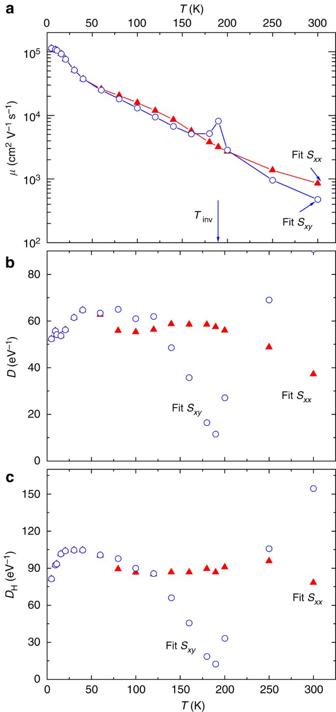Figure 6: Variation of fit parameters versus temperature. TheTdependence of the parametersμ(a), (b) andH(c) obtained from best fits to the curves ofSxx(solid triangles) andSxy(open circles). The fits are most reliable below 100 K where the values obtained from fittingSxxandSxyare in agreement. Above 100 K, disagreement between the two sets is significant, especially close toTinv=180 K. Above 200 K, the one-band model is no longer valid. Figure 6: Variation of fit parameters versus temperature. The T dependence of the parameters μ ( a ), ( b ) and H ( c ) obtained from best fits to the curves of S xx (solid triangles) and S xy (open circles). The fits are most reliable below 100 K where the values obtained from fitting S xx and S xy are in agreement. Above 100 K, disagreement between the two sets is significant, especially close to T inv =180 K. Above 200 K, the one-band model is no longer valid. Full size image Below 100 K, the two sets agree well, whereas closer to T inv they begin to deviate. The reason is that equation 2 cannot account for the change of sign in the Nernst signal given the relative magnitudes of and H fixed by the curves of S xx . Above 200 K, the two sets are inconsistent because thermal excitations of holes across the small band gap is important at elevated T and the one-band assumption becomes inadequate. This is evident in the onset above 200 K of significant T dependence in the Hall density n H (see Fig. 2a ). We remark that S xx = V x /δ T is directly obtained from the observed voltage difference V x and the temperature difference δT between longitudinal electrical contacts (their spatial separation L x is immaterial). However, for the Nernst signal, we have S xy =( V y /δ T )( L x / L y ), where L y is the spatial separation between the transverse contacts. Hence, the aspect ratio L y / L x is needed to convert the observed Nernst voltage V y to S xy . The ratio L y / L x is measured to be 4±0.4. The fits are improved significantly if this value is refined to 4.20, which we adopt for the curves at all T . Fits to equation 9 and 10 of the conductivity tensor measured in the same sample are shown in Fig. 7 for weak B at selected T from 5 to 150 K. The fits yield values of the mobility μ similar to those shown in Fig. 6a . The inferred carrier density N e is also similar to the measured Hall density n H . 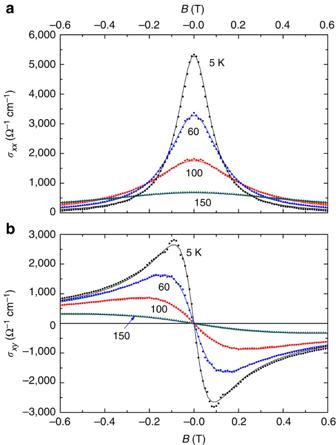Figure 7: Fits of the conductivity tensor. The measured weak-Bconductivityσxx(a) and Hall conductivityσxy(b) of Pb1−xSnxSe (x=0.23) versusBat selectedTfrom 5 to 150 K, together with the fits to equation 9 and 10 (thin solid curves). Figure 7: Fits of the conductivity tensor. The measured weak- B conductivity σ xx ( a ) and Hall conductivity σ xy ( b ) of Pb 1− x Sn x Se ( x =0.23) versus B at selected T from 5 to 150 K, together with the fits to equation 9 and 10 (thin solid curves). Full size image Indexing the quantum oscillations For the 3D systems, one identifies the index field B n as the field at which the DOS displays a sharp maximum (diverging as in the absence of disorder). From the quantization rule for areas in k -space, B n is related to the FS cross-section F as where and γ (the Onsager phase) is for Schödinger electrons. The plot in Fig. 3b follows equation 11. From its slope, we obtain F . The intercept γ is close to zero in Fig. 3b . We will discuss γ elsewhere. We note that, in the 2D systems in the QHE regime, the index field is the field at which the chemical potential ζ falls between adjacent LLs, where the DOS vanishes, and the Hall conductance displays a plateau. The difference between 2D and 3D systems arises because the integer n counts the number of edge states in the QHE case, whereas n indexes the DOS peaks in the 3D case. One needs to keep this in mind in interpreting γ . We have verified that the slope in Fig. 4b is insensitive to the tilt angle θ of B relative to the crystalline axes. As shown in Fig. 5a , the SdH period is virtually independent of θ within the experimental uncertainties, consistent with negligible anisotropy in the small FS pockets. The good agreement between F and n H (Hall density) at 5 K is also evidence for a negligible anisotropy. Spin degeneracy in N =0 LL Knowledge of the field B 1 (the transition from N =1 to the N =0 LL) and the electron density per valley n e suffices to determine the spin degeneracy of the N =0 LL. For the 3D Dirac case [24] , the energy in the N th LL is with m D the Dirac mass, k z the component of k along B and the magnetic length. For N =0 LL, we solve for k z ( E ) where E 00 = m D v 2 . Let us assume that only N =0 LL is occupied. To obtain the relation linking E F , B and n e , we integrate the 3D DOS ( E ) dE =( g L g s / π ) dk z , with g s the spin degeneracy and the 2D LL degeneracy per spin. Using equation 13, we have This equation is valid until B is reduced to the jump field B 1 , whereafter electrons enter the N =1 LL. At the jump field, E F lies just below the bottom of N =1 LL, that is, . Using this in equation 14, we have In relation to equation 3, we showed that equation 15 gives a value equal (within 10%) to the total electron density per valley if g s =1, that is, when B > B 1 , all the electrons can be accomodated by the N =0 LL with only one spin polarization. This is direct evidence for the non-degeneracy of the N =0 LL. Interestingly, equation 15 is identical for the isotropic Schrödinger case, for which where ω c = eB / m and m is the mass. However, for N =0 LL of the Schrödinger spectrum, we must have g s =2, so it can be excluded. A simple example of massive Dirac spectrum An example illustrating the non-degeneracy of N =0 LL is the spinless fermion on the 2D hexagonal lattice (valley degeneracy replaces spin degeneracy in this example). The sublattices A and B have distinct on-site energies ε A and ε B as in BN. The Dirac cones remain centred at the inequivalent ‘valleys’ K and K′ in k -space (inset, Fig. 8 ). Both valleys acquire a mass gap. 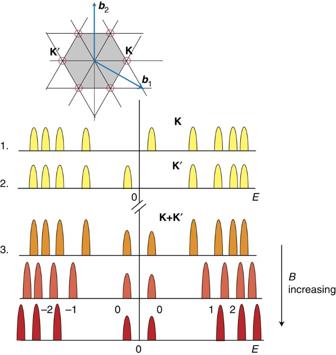Figure 8: The massive Dirac spectrum in the 2D hexagonal lattice. We assume distinct on-site energies on sublattices A and B (as in boron nitride). The Dirac cones sit at the high-symmetry pointsKandK′on the edge of the Brillouin Zone (upper inset). In a magnetic fieldB, theN=0 LL atKmoves to a value aboveE=0 (curve 1), whereas theN=0 LL atK′ moves belowE=0 (curve 2). The sum of the two spectra (K+K′) is symmetric aboutE=0 (curves 3). However, theN=0 LLs are non-degenerate, whereas all other LLs (N≠0) have a valley degeneracy of 2. AsBincreases, all LLs fan out except for theN=0 levels (curves 3). Figure 8: The massive Dirac spectrum in the 2D hexagonal lattice. We assume distinct on-site energies on sublattices A and B (as in boron nitride). The Dirac cones sit at the high-symmetry points K and K′ on the edge of the Brillouin Zone (upper inset). In a magnetic field B , the N =0 LL at K moves to a value above E =0 (curve 1), whereas the N =0 LL at K ′ moves below E =0 (curve 2). The sum of the two spectra ( K+K′ ) is symmetric about E =0 (curves 3). However, the N =0 LLs are non-degenerate, whereas all other LLs ( N ≠0) have a valley degeneracy of 2. As B increases, all LLs fan out except for the N =0 levels (curves 3). Full size image For states close to the valley at K , the 2D massive Dirac Hamiltonian is in the basis (1,0) T (pseudospin up) and (0,1) T (pseudospin down), where k is measured from K and m >0 represents the gap parameter proportional to ε A – ε B (we set the velocity v to 1). In a field B , we replace k by π = k – e A with the vector gauge A =(0, Bx ,0). Introducing the operators with π ± = π x ± iπ y , and eigenstates | N › satisfying we diagonalize the Hamiltonian to get eigenenergies E N given by (for brevity, we will write E for E N ). For positive E , the (unrenormalized) two-spinor eigenstates are (for N =0,1, ⋯ ) For the negative energy states, the corresponding eigenvectors are ( N =1,2, ⋯ ) Setting N =0 in equation 21, we find that the positive-energy state |Ψ 0,+ ›=(|0›,0) T (pseudospin up). For E <0, however, the lower entry in equation 22 is non-determinate (0/0). This implies that the state N =0 does not exist for E <0. Thus, for the valley at K , there is only one LL with N =0. It has positive energy E 0 =| m |; the corresponding LL at −| m | is absent (the spectrum of K is sketched as curve 1 in Fig. 8 ). Repeating the calculation for K′ , we find the opposite situation (the Hamiltonian is the conjugate of equation 17). Now N =0 LL has energy E 0 =−| m |, but N =0 LL is absent in the positive spectrum (the spectrum of K′ is the curve 2 in Fig. 8 ). A transport experiment detects the sum of the two spectra (curves of K+K′ at different B are collectively labelled as 3 in Fig. 8 ). In the total spectrum, the two N =0 LLs are non-degenerate, whereas all LLs with N ≠0 have a valley degeneracy of 2. The difference simply reflects the conservation of states. In the limit m →0, we recover the spectrum of graphene. If, at finite m , each of the N =0 LLs had a valley degeneracy of 2, we would end up with an N =0 LL in graphene with fourfold valley degeneracy. The authors in refs 22 , 23 , 24 and others have shown that the non-degeneracy of the N =0 LL also holds in massive Dirac systems even when a Rashba term and a Zeeman energy term are included. How to cite this article: Liang, T. et al. Evidence for massive bulk Dirac fermions in Pb 1− x Sn x Se from Nernst and thermopower experiments. Nat. Commun. 4:2696 doi: 10.1038/ncomms3696 (2013).